Regulation ofTRI5expression and deoxynivalenol biosynthesis by a long non-coding RNA inFusarium graminearum Deoxynivalenol (DON) is the most frequently detected mycotoxin in cereal grains and processed food or feed. Two transcription factors, Tri6 and Tri10, are essential for DON biosynthesis in Fusarium graminearum . In this study we conduct stranded RNA-seq analysis with tri6 and tri10 mutants and show that Tri10 acts as a master regulator controlling the expression of sense and antisense transcripts of TRI6 and over 450 genes with diverse functions. TRI6 is more specific for regulating TRI genes although it negatively regulates TRI10 . Two other TRI genes, including TRI5 that encodes a key enzyme for DON biosynthesis, also have antisense transcripts. Both Tri6 and Tri10 are essential for TRI5 expression and for suppression of antisense- TRI5 . Furthermore, we identify a long non-coding RNA (named RNA5P) that is transcribed from the TRI5 promoter region and is also regulated by Tri6 and Tri10. Deletion of RNA5P by replacing the promoter region of TRI5 with that of TRI12 increases TRI5 expression and DON biosynthesis, indicating that RNA5P suppresses TRI5 expression. However, ectopic constitutive overexpression of RNA5P has no effect on DON biosynthesis and TRI5 expression. Nevertheless, elevated expression of RNA5P in situ reduces TRI5 expression and DON production. Our results indicate that TRI10 and TRI6 regulate each other’s expression, and both are important for suppressing the expression of RNA5P, a long non-coding RNA with cis -acting inhibitory effects on TRI5 expression and DON biosynthesis in F. graminearum . Fusarium head blight (FHB) is a devastating disease of wheat and barley that threatens global food security. Fusarium graminearum is one major causal agent of FHB and it also infects corn, millets, and other grain crops [1] , [2] , [3] , [4] . In addition to causing significant yield losses, F. graminearum is a producer of deoxynivalenol (DON), which is the most frequently detected mycotoxin in cereal grains and food or feed processed from cereal grains [5] . As a type B trichothecene mycotoxin, DON is inhibitory to eukaryotic protein synthesis and harmful to human or animal health. It is also phytotoxic and DON production plays a critical role during plant infection [6] , [7] . The gene that encodes the Tri5 trichodiene synthase is the first virulence factor functionally characterized by molecular genetic studies in F. graminearum [8] . The tri5 deletion mutant still causes typical symptoms at the inoculated spikelets but fails to spread to neighboring spikelets on the same head via the rachis [9] , [10] . Like in Fusarium sporotrichioides , a producer of type A trichothecene T-2 toxin, the 15 TRI genes related to trichothecene biosynthesis are distributed on three chromosomes in F. graminearum [7] , [11] , [12] , [13] , [14] , [15] . Whereas TRI1-TRI16 and TRI101 are on chromosomes 1 and 3, respectively, the core TRI cluster that contains 12 genes, including TRI5 , TRI6 , and TRI10 , is on chromosome 2 [11] , [13] . The precursor for trichothecene synthesis is farnesyl pyrophosphate (FPP) which is synthesized via the mevalonate pathway [15] , [16] , [17] , [18] . The Tri5 trichodiene synthase catalyzes the first step in trichothecene biosynthesis by cyclizing FPP to trichodiene. The TRI1 , TRI3 , TRI4 , TRI8 , TRI11 , and TRI101 genes encode enzymes responsible for catalyzing the other steps of DON biosynthesis and their expression is under the control of TRI6 and TRI10 [7] , [18] . For the other TRI genes, TRI12 encodes a major facilitator transporter functioning as the trichothecene efflux pump [19] . Whereas the function of TRI9 and TRI14 in trichothecene biosynthesis is not clear [20] , TRI7 , TRI13 , and TRI16 are pseudogenes with frameshift or nonsense mutations in DON-producing strains of F. graminearum [21] , [22] , [23] . In filamentous fungi, gene clusters responsible for the synthesis of secondary metabolites often contain one transcription factor that functions as a pathway-specific regulator of other genes in the same cluster. Interestingly, two of the TRI genes, TRI6 and TRI10 , function as transcriptional regulators of trichothecene biosynthesis in different Fusarium species [7] , [13] . In F. graminearum , both TRI6 and TRI10 are important for TRI gene expression, DON production, and plant infection [18] , [24] . Microarray analysis with infected wheat heads showed that the promoters of most TRI genes and other F. graminearum genes regulated by TRI6 have the YNAGGCC motif [18] , which is similar to the Tri6-binding site reported in F. sporotrichioides [25] . In a later study, a motif of GTGA repeats was identified by ChIP-seq analysis with a TRI6 -HA transformant cultured under nutrient-rich conditions and verified to be recognized by Tri6 proteins in gel mobility shift assays [26] . Unlike Tri6 which is a Cys 2 His 2 zinc finger protein, the Tri10 protein has no DNA-binding domain. Based on microarray analysis, TRI6 expression is not affected in the tri10 deletion mutant although deletion of TRI6 has a minor effect on the expression of TRI10 . Therefore, the mechanism for regulating TRI gene expression by TRI10 and the functional relationship between TRI6 and TRI10 in regulating trichothecene biosynthesis are not clear in F. graminearum . Nevertheless, microarray analysis and qRT-PCR assays used in earlier studies could not distinguish sense and antisense transcripts and are not suitable to characterize the expression levels of TRI genes with antisense transcripts. To better understand the roles of TRI6 and TRI10 in regulating TRI gene expression and DON biosynthesis, in this study, we conducted strand-specific RNA-seq analysis with the tri6 and tri10 deletion mutants under DON-inducing conditions. Although many TRI genes were down-regulated in both mutants, we found that TRI10 regulated the expression of over 450 genes with diverse functions but TRI6 was more specific for regulating TRI genes. As the master regulator, TRI10 was essential for the expression of TRI6 and suppression of antisense- TRI6 . Antisense transcripts of TRI5 and a lncRNA transcribed from its promoter (named RNA5P) also were identified in the tri6 and tri10 mutants. Although overexpression of RNA5P ectopically with the RP27 promoter had no effect, increased expression of RNA5P in situ resulted in a significant reduction or elimination of TRI5 expression and DON production. In contrast, deletion of RNA5P increased DON production and TRI5 expression. Taken together, these results indicate that both TRI10 and TRI6 are important for suppressing the expression of antisense -TRI5 as well as RNA5P, which is a lncRNA inhibitory to TRI5 expression and DON biosynthesis in F. graminearum . TRI10 regulates more genes than TRI6 under DON-inducing conditions Both TRI6 and TRI10 are in the same transcription direction with TRI5 and they are on a 7.5-kb region in the core TRI gene cluster (Fig. 1a ). 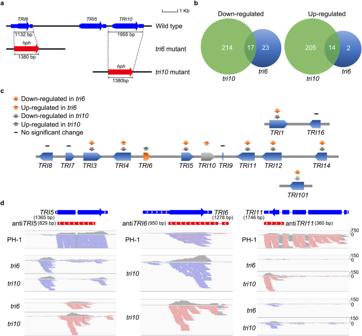Fig. 1: Comparative analysis of DEGs identified in thetri6andtri10mutants. aThe structure of the core trichothecene gene cluster (TRI6-TRI5-TRI10locus) in the wild-type strain PH-1 and gene replacement events in thetri6andtri10deletion mutants. The transcription direction was indicated by the arrow.bVenn diagrams of DEGs down-regulated (left) and up-regulated (right) in thetri6andtri10mutants in comparison with the wild type. Among the 56 DEGs identified in thetri6mutant, 31 (over 55%) were also differentially expressed in thetri10mutant.cSchematic drawing ofTRIgenes and their expression profiles in thetri6andtri10mutants compared to the wild type.dIGV-Sashimi plots showing the read coverage and read counts of sense and anti-sense transcripts ofTRI5,TRI6, andTRI11in the wild type and thetri6andtri10mutants. Schematic draws on the top showed their transcripts and ORFs. The scale on the right indicates the number of read counts. The length of sense and antisense transcripts ofTRI5,TRI6, andTRI11were indicated in the figure. To identify genes regulated by TRI6 and TRI10 , we conducted RNA-seq analysis with the wild type and the tri6 and tri10 mutants [18] (Supplementary Table 1 ) cultured in DON-producing LTB (liquid trichothecene biosynthesis) medium for three days. The tri6 and tri10 mutants we used were generated in a previous study by gene replacement with the hygromycin phosphotransferase ( hph ) cassette (Fig. 1a ). Whereas the TRI5 - TRI6 region was 248-bp longer in the tri6 mutant, the TRI5 - TRI10 region was 575-bp shorter in the tri10 mutant in comparison with the wild type (Fig. 1a ) due to the gene replacement events [18] . In comparison with the wild type, a total of 56 and 450 differentially expressed genes (DEGs) had over 2-fold changes in their expression levels in the tri6 and tri10 mutants, respectively. Among them, 40 and 16 DEGs were down- and up-regulated in the tri6 mutant (Supplementary Data 1 ). In the tri10 mutant, 231 and 219 DEGs were down- and up-regulated, respectively (Supplementary Data 2 ). These results indicate that TRI10 regulates more genes than TRI6 in F. graminearum in DON-producing cultures. GO enrichment analysis showed that DEGs down-regulated in the tri6 mutant are enriched for genes involved in toxin metabolic process and pyridoxal phosphate biosynthesis or metabolism (Supplementary Fig. 1a ). In the tri10 mutant, down-regulated DEGs are enriched for genes associated with RNA transcription, binding, and processing (Supplementary Fig. 1b ). Fig. 1: Comparative analysis of DEGs identified in the tri6 and tri10 mutants. a The structure of the core trichothecene gene cluster ( TRI6 - TRI5 - TRI10 locus) in the wild-type strain PH-1 and gene replacement events in the tri6 and tri10 deletion mutants. The transcription direction was indicated by the arrow. b Venn diagrams of DEGs down-regulated (left) and up-regulated (right) in the tri6 and tri10 mutants in comparison with the wild type. Among the 56 DEGs identified in the tri6 mutant, 31 (over 55%) were also differentially expressed in the tri10 mutant. c Schematic drawing of TRI genes and their expression profiles in the tri6 and tri10 mutants compared to the wild type. d IGV-Sashimi plots showing the read coverage and read counts of sense and anti-sense transcripts of TRI5 , TRI6 , and TRI11 in the wild type and the tri6 and tri10 mutants. Schematic draws on the top showed their transcripts and ORFs. The scale on the right indicates the number of read counts. The length of sense and antisense transcripts of TRI5 , TRI6 , and TRI11 were indicated in the figure. Full size image We then compared RNA-seq data of the tri6 and tri10 mutants and found that 17 and 14 DEGs were down- or up-regulated in both mutants (Fig. 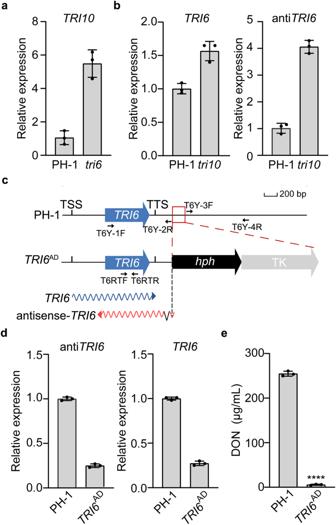Fig. 2: Regulation ofTRI6expression byTRI10and vice versa. aRelative expression levels ofTRI10in 3-day-old LTB cultures of the wild-type strain PH-1 (arbitrarily set to 1) andtri6mutant were assayed by qRT-PCR with primers amplified the 3’-terminal region ofTRI10.bRelative expression levels ofTRI6and antisense-TRI6in PH-1 (arbitrarily set to 1) and thetri10mutant were assayed with strand-specific qRT-PCR. Deletion ofTRI10significantly increased the transcription of antisense-TRI6.cSchematic drawing of theTRI6ORF and its sense or antisense transcripts. In theTRI6ADmutant allele, the 185-bp promoter region (red box) was replaced with the hygromycin phosphotransferase (hph) fusion with thymidine kinase (TK) genes. TSS/TTS, transcription start/termination site. Fragments were amplified with the primer pairs T6Y-1F/ T6Y-2R and T6Y-3F/T6Y-4R for the generation of theTRI6ADstrain, and the primer pair T6RTF/T6RTR was used for qRT-PCR assay.dRelative expression levels ofTRI6and antisense-TRI6in 3-day-old LTB cultures of PH-1 andTRI6ADmutant.eDON production in 7-day-old LTB cultures of PH-1 and theTRI6ADmutants. Fora,b,dande, mean and standard deviation were estimated with data from three (n= 3) independent replicates (marked with black dots on the bars). For DON production, the statistical difference relative to PH-1 is based on the two-tailed unpairedttest (****,p< 0.0001). The exactp-values are shown in the Source Data file. 1b and Supplementary Table 2 ). A total of 7 TRI genes were down-regulated in both mutants (Fig. 1c ), indicating positive regulation by both TRI6 and TRI10 . Among the four TRI genes without significant changes in expression levels in the tri6 or tri10 mutant (Fig. 1c ), TRI7 , TRI13 , and TRI16 are pseudogenes with frameshift and nonsense mutations in DON-producing strains of F. graminearum such as PH-1 [21] , [22] , [23] . For TRI8 which encodes a trichothecene 3-O-esterase, its expression was reduced but less than 2-fold in the tri6 or tri10 mutant. Interestingly, among the 230 DEGs down-regulated in the tri10 mutant, only TRI4 was a DEG up-regulated in the tri6 mutant (Fig. 1c ). Because TRI4 shares the same promoter region with TRI6 , up-regulated expression of TRI4 expression in the tri6 mutant may be directly related to the abolishment of the self-inhibitory binding of Tri6 to its own promoter [26] . To evaluate the potential effects of hph cassette transcription on neighboring TRI genes, we generated the tri6 and tri10 deletion mutants with the hph cassette transcribed in the opposite direction from TRI5 and TRI6 or TRI10 (Supplementary Fig. 2a, b ). The resulting tri6 and tri10 deletion mutants had the same defects in TRI5 expression and DON biosynthesis with the published mutants [18] (Supplementary Fig. 2c–e ), indicating that the TRI6 and TRI10 gene deletion events but not the direction of hph are responsible for the defects observed in the tri6 and tri10 mutants. Expression of antisense transcripts of TRI5 , TRI6 , and TRI11 in the tri6 or tri10 mutant Because our data were generated by stranded RNA-seq, we then separated the sense and antisense transcripts of the TRI genes and examined for changes in their abundance in the tri6 and tri10 mutants compared to the wild type. 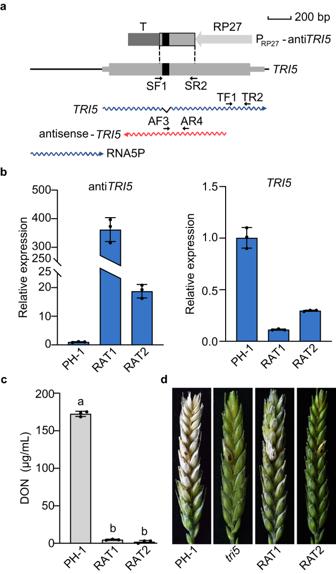Fig. 3: Overexpression of antisense-TRI5inhibits DON biosynthesis. aSchematic drawing of theTRI5ORF, its sense or antisense transcripts, and lncRNA RNA5P as well as the PRP27-antiTRI5construct in which a 299-bp fragment was cloned between the RP27 promoter (RP27) and CaMV ployA signal terminator (T). The black box marks the intron ofTRI5. Arrows indicate the position and orientation of the primers. The fragment was amplified with the primer pair SF1/SR2 for the generation of the PRP27-antiTRI5construct, and the primer pairs TF1/TR2 and AF3/AF4 were used to assay the expression ofTRI5and antisense-TRI5, respectively.bRelative expression levels of antisense-TRI5andTRI5in 3-day-old LTB cultures of the wild type (PH-1) and PRP27-antiTRI5transformant (RAT1 and RAT2). The relative expression level in PH-1 was arbitrarily set to 1.cDON production in 7-day-old LTB cultures of PH-1 and PRP27-antiTRI5(RAT1 and RAT2).dWheat heads inoculated with the indicated strains were examined for head blight symptoms at 14 days post-inoculation (dpi). Black dots mark the inoculated spikelets. Forbandc, mean and standard deviation were estimated with data from three (n= 3) independent replicates (marked with black dots on the bars). For DON production, different letters indicate significant differences based on the one-way ANOVA followed by Turkey’s multiple range test. Differences were considered statistically significant whenp-value is <0.05. The exactp-values are shown in the Source Data file. In the wild type, only TRI5 and TRI6 had rare anti-sense transcripts (Supplementary Table 3 ). In the tri10 mutant, antisense transcripts of TRI5 and TRI6 were significantly increased (Fig. 1d ). For the TRI5 gene, sense transcripts were rare but antisense transcripts were abundant in the tri6 and tri10 mutants (Fig. 1d ), indicating a negative regulation of antisense- TRI5 by TRI6 and TRI10 . For TRI11 , the only other TRI genes with antisense transcripts detected in this study, its sense transcripts were rare in the tri6 and tri10 mutants, a significant reduction compared to the wild type. Antisense transcripts of TRI11 were present in both mutants but more abundant in the tri10 mutant (Fig. 1d ). These results indicate that TRI6 and TRI10 are not only essential for the expression of sense transcripts of TRI5 and TRI11 but also important for suppressing their antisense transcription. Based on the stranded RNA-seq data, antisense transcripts of the other TRI genes were not detected in the wild type, and the tri6 and tri10 mutants (Supplementary Fig. 3 ). Repression of TRI10 expression by TRI6 and vice versa TRI10 has no antisense transcripts in the wild type and tri6 mutant. However, the expression level of TRI10 was significantly increased (over 2-fold) in the tri6 mutant compared to the wild type (Fig. 2a ). These results indicate that TRI10 expression is negatively regulated by TRI6 . In the tri10 deletion mutant, the expression level of antisense- TRI6 was significantly increased (over 4-fold) based on both RNA-seq (Fig. 1d ) and qRT-PCR assays (Fig. 2b ) compared to the wild type. For the sense transcripts of TRI6 , the overall abundance was also increased in the tri10 mutant due to a significant increase in partial transcripts mapped to the 3’-terminal region of TRI6 (Fig. 1d ; Fig. 2b ). Close examination showed that antisense transcripts of TRI6 predominantly mapped to its 5’-terminal 410-bp region. In contrast, the 3’-terminal 274-bp region of TRI6 was more abundant in its sense transcripts (Fig. 1d ), suggesting the pairing and degradation of TRI6 mRNA by antisense- TRI6 transcripts. These results indicate that the expression of sense and antisense transcripts of TRI6 , is negatively regulated by TRI10 . Interestingly, antisense transcripts mapped to the terminator region of TRI6 had a 65-bp intron (Fig. 1d ) that is a part of antisense- TRI6 based on RT-PCR assays (Supplementary Fig. 4a, b ). To test the importance of this intron, we generated the TRI6 ME mutant allele, in which the GT-AG splicing sites were changed to AT-TG, and transformed into the tri6 mutant (Supplementary Fig. 4a, b ). In LTB cultures, the resulting tri6 / TRI6 ME transformant was normal in DON biosynthesis and TRI6 expression (Supplementary Fig. 4c, d ), indicating that splicing of this intron in antisense transcripts is not important for the function of TRI6 . Fig. 2: Regulation of TRI6 expression by TRI10 and vice versa. a Relative expression levels of TRI10 in 3-day-old LTB cultures of the wild-type strain PH-1 (arbitrarily set to 1) and tri6 mutant were assayed by qRT-PCR with primers amplified the 3’-terminal region of TRI10 . b Relative expression levels of TRI6 and antisense- TRI6 in PH-1 (arbitrarily set to 1) and the tri10 mutant were assayed with strand-specific qRT-PCR. Deletion of TRI10 significantly increased the transcription of antisense- TRI6 . c Schematic drawing of the TRI6 ORF and its sense or antisense transcripts. In the TRI6 AD mutant allele, the 185-bp promoter region (red box) was replaced with the hygromycin phosphotransferase ( hph ) fusion with thymidine kinase (TK) genes. TSS/TTS, transcription start/termination site. Fragments were amplified with the primer pairs T6Y-1F/ T6Y-2R and T6Y-3F/T6Y-4R for the generation of the TRI6 AD strain, and the primer pair T6RTF/T6RTR was used for qRT-PCR assay. d Relative expression levels of TRI6 and antisense- TRI6 in 3-day-old LTB cultures of PH-1 and TRI6 AD mutant. e DON production in 7-day-old LTB cultures of PH-1 and the TRI6 AD mutants. For a , b , d and e , mean and standard deviation were estimated with data from three ( n = 3) independent replicates (marked with black dots on the bars). For DON production, the statistical difference relative to PH-1 is based on the two-tailed unpaired t test (****, p < 0.0001). The exact p -values are shown in the Source Data file. Full size image We then generated mutants deleted of a 185-bp region covering parts of the terminator region of TRI6 by the gene replacement approach (Fig. 2c ). This region likely contains the promoter region for antisense -TRI6 . In the resulting TRI6 AD transformant (Supplementary Table 1 ), antisense transcripts of TRI6 were significantly reduced in qRT-PCR assays with RNA isolated from LTB cultures (Fig. 2d ). However, the expression of TRI6 sense transcripts and DON production were also significantly reduced in the TRI6 AD mutant (Fig. 2d, e ). Therefore, deletion of this 185-bp region and insertion of the selectable marker at the TRI6 locus likely affect the expression of both sense and antisense transcripts, possibly by interfering with the initiation of their transcription, transcription efficiency, or transcript stability. Overexpression of antisense- TRI5 inhibits DON biosynthesis Antisense transcripts of TRI5 were not detectable in the wild type under DON inducing conditions but were abundant in both tri6 and tri10 mutants. To determine the function of antisense- TRI5 transcripts, we generated the P RP27 -anti TRI5 construct and transformed it into PH-1 (Fig. 3a ). Transformants with the P RP27 -anti TRI5 construct integrated ectopically were isolated (Supplementary Table 1 ) and assayed for TRI5 and DON production in LTB cultures. In comparison with the wild type, the expression of antisense- TRI5 was increased over 20-fold but DON production and the expression level of TRI5 was significantly reduced in the P RP27 -anti TRI5 transformants (Fig. 3b, c ). In plant infection assays, P RP27 -anti TRI5 transformants, like the tri5 mutant, caused symptoms only on the inoculated wheat spikelet (Fig. 3d ). These results indicate that overexpression of antisense- TRI5 reduced the sense transcripts of TRI5 and inhibitory to DON biosynthesis. Fig. 3: Overexpression of antisense- TRI5 inhibits DON biosynthesis. a Schematic drawing of the TRI5 ORF, its sense or antisense transcripts, and lncRNA RNA5P as well as the P RP27 -anti TRI5 construct in which a 299-bp fragment was cloned between the RP27 promoter (RP27) and CaMV ployA signal terminator (T). The black box marks the intron of TRI5 . Arrows indicate the position and orientation of the primers. The fragment was amplified with the primer pair SF1/SR2 for the generation of the P RP27 -anti TRI5 construct, and the primer pairs TF1/TR2 and AF3/AF4 were used to assay the expression of TRI5 and antisense- TRI5 , respectively. b Relative expression levels of antisense- TRI5 and TRI5 in 3-day-old LTB cultures of the wild type (PH-1) and P RP27 -anti TRI5 transformant (RAT1 and RAT2). The relative expression level in PH-1 was arbitrarily set to 1. c DON production in 7-day-old LTB cultures of PH-1 and P RP27 -anti TRI5 (RAT1 and RAT2). d Wheat heads inoculated with the indicated strains were examined for head blight symptoms at 14 days post-inoculation (dpi). Black dots mark the inoculated spikelets. For b and c , mean and standard deviation were estimated with data from three ( n = 3) independent replicates (marked with black dots on the bars). For DON production, different letters indicate significant differences based on the one-way ANOVA followed by Turkey’s multiple range test. Differences were considered statistically significant when p -value is <0.05. The exact p -values are shown in the Source Data file. Full size image RNA5P is a lncRNA mapped to the promoter region of TRI5 Close examination of strand-specific RNA-seq data showed that, under DON-inducing conditions, the 675-bp transcripts mapped to the promoter region of TRI5 (named RNA5P for RNA transcribed from the TRI 5 p romoter) were rare in PH-1 but became abundant in the tri6 and tri10 mutants, especially in the latter (Fig. 1c and Supplementary Table 3 ). Furthermore, RNA5P has one intron that was spliced in a small percentage of RNA5P transcripts in the tri6 and tri10 mutants (Fig. 1c ). Alternative splicing of this intron will lead to two transcripts of RNA5P (Fig. 4a ). Based on prediction with ExPASy (web.expasy.org/translate), these two transcripts may encode two small peptides of 58- and 86-amino acid residues that share the same stop codon (Fig. 4a and Supplementary Fig. 5 ). To test whether RNA5P is a part of TRI5 mRNA, we conducted RT-PCR analysis with RNA isolated from LTB cultures of PH-1. Whereas primer pairs 5PRT1/5PRT2 and TF1/TR2 amplified the 0.11 and 0.18-kb band, respectively, no band could be amplified with primer pairs 5PRT1 and TR2 (Fig. 4b ), indicating that RNA5P transcripts are independent of TRI5 mRNA. Fig. 4: RNA5P is a lncRNA transcribed from the TRI5 promoter. a Schematic drawing of the genomic region of RNA5P, its transcripts, and the P RP27 -RNA5P-3×FLAG fusion construct. Two isoforms of RNA5P (isoform-1 and isoform-2) are formed due to alternative splicing of the intron (black box) and are predicted to encode two small proteins that share the same stop codon. RP27, RP27 promoter; T, CaMV ployA signal terminator; TSS/TTS, transcription start/termination site. b PCR products amplified with primer pairs 5PRT1/5PRT2 (lane 1), TF1/TR2 (lane 2), and 5PRT1/TR2 (lane 3) from genomic DNA and 1 st strand cDNA synthesized with RNA isolated from LTB cultures of the wild-type strain PH-1. M, molecular marker. The experiment was repeated three times independently with similar results. c Relative expression levels of RNA5P in LTB cultures of PH-1 and the P RP27 -RNA5P-3×FLAG transformant. d Western blots of total proteins isolated from transformants expressing the P RP27 -RNA5P-3×FLAG and the FgESA1 -3×FLAG (as the positive control) fusion constructs were detected with the anti-FLAG and anti-Tubulin antibodies. e Schematic drawing of in situ nucleotide insertion in RNA5P. The hph -TK cassette in the TRI5 Δpromoter transformant (T5P) was replaced with a fragment with an adenine (A) insertion in the RNA5P (amplified with labeled primer pairs) by selecting transformants resistant to Floxuridine (RNA5P M ). P, TrpC promoter; T, CaMV ployA signal terminator. f The adenine (A) insertion in the RNA5P was verified by Sanger sequencing of the PCR products. The inserted nucleotide is marked with a red star. g Relative expression levels of TRI5 were assayed by qRT-PCR with RNA isolated from LTB cultures of PH-1 (arbitrarily set to 1) and the RNA5P M strain. h DON production in 7-day-old LTB cultures of the PH-1 and the RNA5P M strain. For c , g , and h , mean and standard deviation were estimated with data from three ( n = 3) independent replicates (marked with black dots on the bars). For DON production, no significant statistical differences were observed based on the two-tailed unpaired t test. The exact p -values are shown in the Source Data file. Full size image To test whether RNA5P transcripts can be translated, we generated the RNA5P-3×FLAG fusion construct (Fig. 4a ) under the control of the constitutive RP27 promoter [27] and transformed it into PH-1. In the resulting P RP27 -RNA5P-3×FLAG transformants, the expression of RNA5P was increased in transformants with the fusion construct compared with PH-1 (Fig. 4c ). However, the anti-FLAG antibody failed to detect any band on western blots of total proteins isolated from the resulting RNA5P-3×FLAG transformants cultured in LTB (Fig. 4d ). As the control, the expression of FgEsa1 histone acetyltransferase was detected in the FgESA1 -3xFLAG transformant [28] under the same experimental conditions (Fig. 4d ). To further prove the function of RNA5P is independent of protein coding, we inserted an adenine (A) in the predicted ORF of RNA5P in situ (Fig. 4e and Supplementary Fig. 6 ). The resulting transformant with the frameshift mutation verified by sequencing analysis (Fig. 4f ) was normal in TRI5 expression (Fig. 4g ) and DON production (Fig. 4h ) in comparison with the wild type. These results suggest that RNA5P does not encode functional proteins and likely acts as a lncRNA in F. graminearum . Deletion of RNA5P by promoter switching increases TRI5 expression To characterize the function of RNA5P, we used the gene replacement approach to replace 834-bp region upstream from the TRI5 ORF that contains the RNA5P region with an 834-bp fragment of the TRI12 promoter (Fig. 5a, b ). TRI12 was selected because, like TRI5 , its expression is regulated by both TRI6 and TRI10 but its expression level was 10-fold lower than that of TRI5 based on our RNA-seq data (Fig. 5a, b ). The size of the promoter regions used for promoter swapping was kept similar to avoid possible effects of size changes on local chromatin structures in the TRI gene cluster [14] . In the resulting P TRI12 - TRI5 transformants, the replacement of TRI5 promoter with that of TRI12 was verified by PCR amplification (Supplementary Fig. 7 ). When assayed by qRT-PCR with RNA isolated from LTB cultures, the expression of RNA5P was detected in the wild type but not in the P TRI12 - TRI5 transformant (Fig. 5c ). The expression level of TRI5 sense transcripts was increased 2.6-fold in the P TRI12 - TRI5 transformant compared to the wild type (Fig. 5c ). However, the transcription of antisense- TRI5 was only slightly increased in the P TRI12 - TRI5 transformant (Fig. 5c ). Consistent with increased expression of TRI5 , DON production was also increased in the P TRI12 - TRI5 transformant (Fig. 5d ). Microscopical examination also showed a slight increase in the formation of hyphal swelling or cellular differentiation associated with DON production (Fig. 5e ). These results indicate that even though TRI12 has a lower expression level than TRI5 , deletion of RNA5P by replacing the promoter of TRI5 with that of TRI12 had no significant effect on antisense- TRI5 expression but significantly increased TRI5 expression and DON biosynthesis. Fig. 5: Deletion of RNA5P increase TRI5 expression and DON production. a Expression levels of TRI5 and TRI12 in the LTB cultures of the wild type based on RNA-seq data. b Schematic drawing of in situ replacement of the TRI5 promoter with the TRI12 promoter. The hygromycin phosphotransferase ( hph )-thymidine kinase (TK) cassette in the TRI5 Δpromoter transformant (T5P) was replaced with the TRI12 promoter (amplified with labeled primer pairs) by selecting transformants resistant to Floxuridine (PT12). P, TrpC promoter; T, CaMV ployA signal terminator. c Relative expression levels of RNA5P, TRI5 , and antisense- TRI5 were assayed by qRT-PCR with RNA isolated from LTB cultures of PH-1 (arbitrarily set to 1) and the P TRI12 - TRI5 transformant PT12. d DON production in 7-day-old LTB cultures of the marked strains. e LTB cultures of PH-1 and P TRI12 - TRI5 transformant PT12 were examined for bulbous structures (marked with arrows) related to DON production. Bar = 20 μm. For a , c , and d , mean and standard deviation were estimated with data from three ( n = 3) independent replicates (marked with black dots on the bars). For DON production, the statistical difference relative to PH-1 is based on the two-tailed unpaired t test (*, p < 0.05). The exact p -values are shown in the Source Data file. Full size image Overexpression of RNA5P ectopically has no inhibitory effect on TRI5 expression and DON biosynthesis To determine the effect of RNA5P overexpression, we generated the P RP27 -RNA5P construct (Fig. 6a ) and transformed it into PH-1. In the resulting transformants (Supplementary Table 1 ) the transforming P RP27 -RNA5P construct was ectopically integrated into the wild-type strain PH-1 (Fig. 6a ). The P RP27 -RNA5P transformants (LT7 and LT10) were normal in growth, conidiation, and sexual reproduction (Fig. 6b ). In comparison with the wild type, the expression level of RNA5P was increased over 5-fold in LTB cultures in the P RP27 -RNA5P transformants (Fig. 6c ). However, the expression level of TRI5 (Fig. 6c ) and DON production (Fig. 6d ) were not significantly affected in P RP27 -RNA5P transformants. These results indicate that overexpression of RNA5P ectopically has no inhibitory effects on TRI5 expression and DON biosynthesis. Therefore, the inhibitory effect of RNA5P on TRI5 appears to be cis -acting and require its transcription from the TRI5 locus. Fig. 6: Overexpression of RNA5P has no effect on TRI5 expression and DON production. a Schematic drawing of RNA5P upstream of TRI5 and the generation of P RP27 -RNA5P construct. RP27, PR27 promoter; T, CaMV polyA signal terminator. LT7 and LT10 are two independent transformants with the integration of P RP27 -RNA5P ectopically. UKG, Unknown gene. b Mating cultures of PH-1 and P RP27 -RNA5P transformants (LT7 and LT10) were examined for perithecium formation at 7 days post-fertilization (dpf). 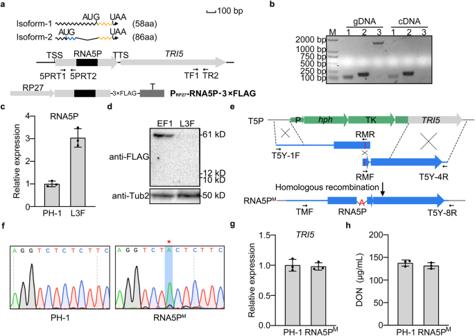Fig. 4: RNA5P is a lncRNA transcribed from theTRI5promoter. aSchematic drawing of the genomic region of RNA5P, its transcripts, and the PRP27-RNA5P-3×FLAG fusion construct. Two isoforms of RNA5P (isoform-1 and isoform-2) are formed due to alternative splicing of the intron (black box) and are predicted to encode two small proteins that share the same stop codon. RP27, RP27 promoter; T, CaMV ployA signal terminator; TSS/TTS, transcription start/termination site.bPCR products amplified with primer pairs 5PRT1/5PRT2 (lane 1), TF1/TR2 (lane 2), and 5PRT1/TR2 (lane 3) from genomic DNA and 1ststrand cDNA synthesized with RNA isolated from LTB cultures of the wild-type strain PH-1. M, molecular marker. The experiment was repeated three times independently with similar results.cRelative expression levels of RNA5P in LTB cultures of PH-1 and the PRP27-RNA5P-3×FLAG transformant.dWestern blots of total proteins isolated from transformants expressing the PRP27-RNA5P-3×FLAG and theFgESA1-3×FLAG (as the positive control) fusion constructs were detected with the anti-FLAG and anti-Tubulin antibodies.eSchematic drawing of in situ nucleotide insertion in RNA5P. Thehph-TK cassette in theTRI5Δpromotertransformant (T5P) was replaced with a fragment with an adenine (A) insertion in the RNA5P (amplified with labeled primer pairs) by selecting transformants resistant to Floxuridine (RNA5PM). P, TrpC promoter; T, CaMV ployA signal terminator.fThe adenine (A) insertion in the RNA5P was verified by Sanger sequencing of the PCR products. The inserted nucleotide is marked with a red star.gRelative expression levels ofTRI5were assayed by qRT-PCR with RNA isolated from LTB cultures of PH-1 (arbitrarily set to 1) and the RNA5PMstrain.hDON production in 7-day-old LTB cultures of the PH-1 and the RNA5PMstrain. Forc,g, andh, mean and standard deviation were estimated with data from three (n= 3) independent replicates (marked with black dots on the bars). For DON production, no significant statistical differences were observed based on the two-tailed unpairedttest. The exactp-values are shown in the Source Data file. Asci and ascospores were examined by DIC microscopy. Bar = 20 μm. c Relative expression levels of RNA5P, TRI5 , and antisense- TRI5 were assayed by qRT-PCR with RNA isolated from LTB cultures of PH-1 (arbitrarily set to 1) and P RP27 -RNA5P transformants (LT7 and LT10). d DON production in 7-day-old LTB cultures of the same set of strains. For c and d , mean and standard deviation were estimated with data from three ( n = 3) independent replicates (marked with black dots on the bars). For DON production, no significant statistical differences were observed based on the one-way ANOVA followed by Turkey’s multiple range test. Differences were considered statistically significant when p -value is <0.05. The exact p -values are shown in the Source Data file. Full size image In situ overexpression of RNA5P with the TrpC promoter suppresses TRI5 expression and DON production To assay the effect of in situ RNA5P overexpression, a 366-bp fragment of the TrpC promoter was inserted 622-bp upstream from the transcription initiation site of RNA5P (126-bp downstream from the predicted Tri6-binding site) by homologous recombination (Fig. 7a ). The integration of the TrpC promoter in the promoter region of RNA5P was verified by PCR amplification (Fig. 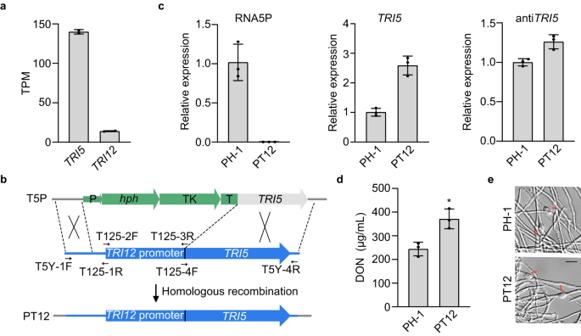Fig. 5: Deletion of RNA5P increaseTRI5expression and DON production. aExpression levels ofTRI5andTRI12in the LTB cultures of the wild type based on RNA-seq data.bSchematic drawing of in situ replacement of theTRI5promoter with theTRI12promoter. The hygromycin phosphotransferase (hph)-thymidine kinase (TK) cassette in theTRI5Δpromotertransformant (T5P) was replaced with theTRI12promoter (amplified with labeled primer pairs) by selecting transformants resistant to Floxuridine (PT12). P, TrpC promoter; T, CaMV ployA signal terminator.cRelative expression levels of RNA5P,TRI5, and antisense-TRI5were assayed by qRT-PCR with RNA isolated from LTB cultures of PH-1 (arbitrarily set to 1) and the PTRI12-TRI5transformant PT12.dDON production in 7-day-old LTB cultures of the marked strains.eLTB cultures of PH-1 and PTRI12-TRI5transformant PT12 were examined for bulbous structures (marked with arrows) related to DON production. Bar = 20 μm. Fora,c, andd, mean and standard deviation were estimated with data from three (n= 3) independent replicates (marked with black dots on the bars). For DON production, the statistical difference relative to PH-1 is based on the two-tailed unpairedttest (*,p< 0.05). The exactp-values are shown in the Source Data file. 7a ). The P TrpC -RNA5P transformants (TR1 and TR2) were normal in growth (Fig. 7b ). In LTB cultures, the expression level of RNA5P was almost 15-fold higher in the P TrpC -RNA5P transformant than in the wild type (Fig. 7c ), indicating increased expression of RNA5P by the TrpC promoter. Fig. 7: In situ overexpression of RNA5P with the TrpC promoter inhibits TRI5 expression. a Insertion of the TrpC promoter in the forward and reverse directions upstream from RNA5P. Red box marks the Tri6-binding site (left panel). PCR products amplified with primer pairs TR-3F/T5Y-8R and ATR-3F/T5Y-8R from genomic DNA of the wild-type strain PH-1, TRI5 Δpromoter transformant (T5P), and the resulting transformants (right panel). The TrpC promoter was successfully inserted upstream of the RNA5P to generate the resulting transformants TR1 and TR2, and the insertion of TrpC-inverted promoter upstream of the RNA5P was verified by PCR in the transformants ATR1 and ATR3. Genomic DNA isolated from the wild-type PH-1 and T5P was used as a control. M, molecular marker. The experiment was repeated three times independently with similar results. b Three days PDA cultures of the wild type (PH-1), P TrpC -RNA5P mutants (TR1 and TR2), and P TrpC-inverted transformants (ATR1 and ATR3). c Relative expression levels of RNA5P, TRI5 , and antisense- TRI5 were assayed by qRT-PCR with RNA samples isolated from LTB cultures of the wild type (PH-1), P TrpC -RNA5P mutants (TR1 and TR2), and P TrpC -Inverted-RNA5P transformants (ATR1 and ATR3). The relative expression level in PH-1 was arbitrarily set to 1. d DON production in LTB cultures of the same set of strains. For c and d , mean and standard deviation were estimated with data from three ( n = 3) independent replicates (marked with black dots on the bars). For DON production, different letters indicate significant differences based on one-way ANOVA followed by Turkey’s multiple-range test. Differences were considered statistically significant when p -value is <0.05. The exact p -values are shown in the Source Data file. Full size image We then assayed TRI5 expression and DON production in LTB cultures. In comparison with the wild type, the expression level of TRI5 was significantly reduced in the P TrpC -RNA5P transformants (Fig. 7c ). DON production was almost non-detectable in the P TrpC -RNA5P mutants (Fig. 7d ). As a control, we also generated transformants with the TrpC promoter sequence integrated at the same site but in the opposite direction (Fig. 7a ). Unlike the P TrpC -RNA5P transformants, the resulting P TrpC-inverted -RNA5P transformants (ATR1 and ATR3) were similar with the wild type in the expression levels of RNA5P and TRI5 (Fig. 7c ) as well as DON biosynthesis (Fig. 7d ). These results indicate that in situ overexpression of RNA5P by the TrpC promoter negatively impacts TRI5 expression and DON biosynthesis, confirming the cis -acting inhibitory effect of RNA5P. Elevated expression of RNA5P by the GTGA to TGAG mutation in its promoter also suppresses DON biosynthesis To confirm the cis -acting effect of RNA5P, we introduced the GTGA (underlined) to TGAG mutation to the TCACGGGCTACA GTGA ATGTTCGTGA sequence found at 748-bp upstream from its transcription initial site. This sequence contains two putative Tri6-binding sites [26] that overlap at the underlined GTGA (Fig. 8a ). In the TRI5 M6B transformants TM6 and TM66 in which the change of underlined GTGA to TGAG was confirmed by PCR amplification and sequencing (Fig. 8b ), the expression level of RNA5P was significantly increased in the TRI5 M6B transformants compared to the wild type in LTB cultures (Fig. 8c ). In comparison with the wild type, the TRI5 M6B transformants were significantly reduced in the expression level of TRI5 (Fig. 8c ) and DON production (Fig. 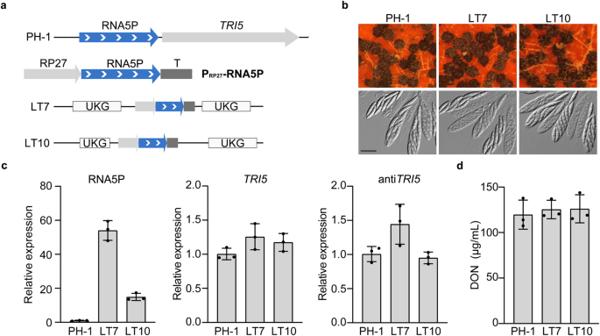Fig. 6: Overexpression of RNA5P has no effect onTRI5expression and DON production. aSchematic drawing of RNA5P upstream ofTRI5and the generation of PRP27-RNA5P construct. RP27, PR27 promoter; T, CaMV polyA signal terminator. LT7 and LT10 are two independent transformants with the integration of PRP27-RNA5P ectopically. UKG, Unknown gene.bMating cultures of PH-1 and PRP27-RNA5P transformants (LT7 and LT10) were examined for perithecium formation at 7 days post-fertilization (dpf). Asci and ascospores were examined by DIC microscopy. Bar = 20 μm.cRelative expression levels of RNA5P,TRI5, and antisense-TRI5were assayed by qRT-PCR with RNA isolated from LTB cultures of PH-1 (arbitrarily set to 1) and PRP27-RNA5P transformants (LT7 and LT10).dDON production in 7-day-old LTB cultures of the same set of strains. Forcandd, mean and standard deviation were estimated with data from three (n= 3) independent replicates (marked with black dots on the bars). For DON production, no significant statistical differences were observed based on the one-way ANOVA followed by Turkey’s multiple range test. Differences were considered statistically significant whenp-value is <0.05. The exactp-values are shown in the Source Data file. 8d ). These results suggest that like the self-inhibitory binding of Tri6 to its own promoter [26] , binding of Tri6 to this GTGA repeat site is suppressive to the expression of RNA5P. Overexpression of RNA5P in situ by the GTGA to TGAG mutation that eliminates the inhibitory binding of Tri6 to its promoter is repressive to TRI5 expression and DON production, confirming the cis -acting effect of RNA5P (Fig. 8e ). Fig. 8: The GTGA to TGAG mutation in the promoter of RNA5P affects its expression and DON biosynthesis. a Schematic drawing of the genomic region of RNA5P and the gene replacement event to introduce the GTGA (underlined) to TGAG mutation at the Tri6-binding site in its promoter. The overlapping PCR products amplified with labeled PCR primers containing the TCACGGGCTACA TGAG ATGTTCGTGA sequence were transformed into the TRI5 Δpromoter transformant (T5P) to generate the TRI5 M6B transformants carrying the GTGA to TGAG mutation. P, TrpC promoter; T, CaMV ployA signal terminator. b The expected sizes of fragments could be amplified with primer pairs T5P-F and T5Y-8R from genomic DNA of the wild type and two independent TRI5 M6B transformants (TM6 and TM66), but not the T5P strain (upper panel). M, molecular marker. The GTGA-to-TGAG mutation in TM6 and TM66 strains was verified by Sanger sequencing of the PCR products (lower panel). The mutations are marked with red stars. The experiment was repeated three times independently with similar results. c Relative expression levels of RNA5P, TRI5 , and antisense- TRI5 in LTB cultures of PH-1 (arbitrarily set to 1) and two independent TRI5 M6B transformants (TM6 and TM66) carrying the GTGA to TGAG mutation. d DON production in LTB cultures of PH-1 and two independent TRI5 M6B transformants (TM6 and TM66). e A proposed model for the role of Tri6-binding on RNA5P expression. In the wild type, binding of Tri6 is inhibitory to RNA5P expression, leading to TRI5 expression under DON-producing conditions. In the mutant with the GTGA-to-TGAG mutation that eliminates Tri6-binding, elevated RNA5P expression results in the suppression of TRI5 expression. For c and d , mean and standard deviation were estimated with data from three ( n = 3) independent replicates (marked with black dots on the bars). For DON production, different letters indicate significant differences based on one-way ANOVA followed by Turkey’s multiple-range test. Differences were considered statistically significant when p -value is <0.05. The exact p -values are shown in the Source Data file. Full size image As an important virulence factor, DON biosynthesis plays a critical role in plant infection in F. graminearum . Similar to earlier studies [18] , our RNA-seq data showed that both TRI6 and TRI10 are required for the expression of many TRI genes essential for DON biosynthesis. However, microarray analysis with the tri6 and tri10 mutants showed that TRI10 is a pathway-specific regulator while TRI6 functions as a regulator to regulate other genes functionally related to plant infection [18] . In this study, we found that deletion of TRI6 only impacted the expression of 56 genes, which was significantly fewer than 450 DEGs in the tri10 mutant. One likely explanation for these contrasting observations is that, although the same strain was used, conditions for RNA isolate was different. For microarray analysis, RNA was isolated from infected wheat heads [18] . In this study, RNA used for RNA-seq analysis was isolated from LTB cultures. It is possible that TRI6 regulates more genes related to plant infection but TRI10 regulates many more genes than TRI6 in DON-producing, axenic cultures. In F. graminearum , differences in TRI gene regulation exist between planta and cultures. In F. graminearum , differences in DON biosynthesis between axenic cultures and infected plant tissues have been observed in mutants deleted of TRI14 that encodes a hypothetical protein of no known functions [20] . In F. sporotrichioides , TRI10 functions as the principal regulatory element, orchestrating the expression of TRI6 . While TRI10 regulates many other genes, TRI6 exhibits a more specific role in governing the TRI genes associated with T-2 toxin production [29] , [30] , which is similar to what we observed in F. graminearum . Because sense transcripts are not distinguished from antisense transcripts by conventional microarray analysis and qRT-PCR assays, deletion of TRI10 seemingly displayed no obvious effect on TRI6 expression as shown by Seong and colleagues [18] . In this study, we found that TRI6 is one of the three TRI genes with antisense transcripts. In comparison with the wild type, antisense transcripts of TRI6 in the tri10 mutant became more abundant as detected by microarray analysis and qRT-PCR assays [18] . For TRI10 , it had no antisense transcripts, and its expression was increased over 5-fold in the tri6 mutant, which is similar to the negative regulation of TRI10 by TRI6 in F. sporotrichioides [29] . Therefore, TRI6 and TRI10 may regulate each other’s expression in LTB cultures with TRI10 is the master, global regulator in F. graminearum . Because TRI6 expression is regulated by TRI10 and lacks any known DNA-binding domain, it is possible that regulation of other TRI genes by TRI10 is mediated by TRI6 . In concordance, TRI6 was reported to interact with pathway-specific transcription factor Gra2 for the regulation of gramillin biosynthesis [31] . TRI10 may also regulate different subsets of genes by interacting with pathway-specific transcription factors. Interestingly, a recent study with the Tri6_nsm mutant carrying a nonsense mutation in TRI6 (no changes in the length of TRI6 ) and Δ Tri6 tk gene replacement mutant (with an increase of 7.0-kp at the TRI6 locus) showed that the expression of TRI10 was elevated in the latter but not in the Tri6 _ nsm mutant [14] , suggesting a possible effect of changes in the length of TRI6 and regional chromatin structures on TRI10 expression. Unlike the 7.0-kb increase the Δ Tri6 tk strain, the gene replacement event in the tri6 mutant resulted an increase of only 248-bp at the TRI6 locus [18] , which is 2.6-kp upstream from TRI5 (Fig. 1a ). The defect of the tri6 mutant in DON biosynthesis was largely complemented by ectopic expression of TRI6 [18] confirming that the phenotype observed in the mutant is related to TRI6 deletion. Similarly, the tri10 deletion mutant was complemented by ectopic expression of TRI10 and the gene replacement event at this locus resulted in a shortening of 575-bp [18] . Furthermore, changes in chromatin structures usually create an environment that is permissive for similar activation or repression of neighboring genes [32] , however, the tri6 deletion mutant was significantly reduced in TRI5 expression but increased in TRI10 expression although all three genes in the TRI6-TRI5-TRI10 region are transcribed in the same direction (Fig. 1a ). The opposite effects of TRI6 deletion on the expression of TRI5 and TRI10 further indicate that changes in TRI expression in the tri6 mutant is likely due to its transcriptional regulation by TRI6 . Nevertheless, we noticed differences in culture conditions and F. graminearu m strains used by Liew and colleagues [14] and in this study [18] . Because DON is a secondary metabolite, we normally assay DON production and TRI gene expression in cultures of strain PH-1 [33] that have been incubated for at least for 72 h. It is also noteworthy that the nonsense mutation at the Methionine (Met) residue (A 10 TG 12 to TAG) in the Tri6_nsm mutant of strain JCM 9873 [14] is towards the N-terminus of Tri6 and truncated proteins may be translated from downstream in-frame ATG or CTG/GTG codons [34] . Overall, the regulation on TRI genes is multilayered and involves transcription factors, antisense transcripts, and chromosomal organization. In comparison with the wild type, the expression of antisense- TRI5 was significantly up-regulated in the tri6 and tri10 mutants, suggesting a negative regulation by TRI6 and TRI10 . Because full-length sense transcripts of TRI5 were rare or absent in the tri6 and tri10 mutants, detection of TRI5 expression by qRT-PCR or microarray analysis in both mutants in earlier studies [18] could be due to its antisense transcripts. For the RNA5P lncRNA transcribed from the promoter region of TRI5 , its expression is also negatively regulated by both TRI6 and TRI10 . Because mutations at the GTGA repeats in its promoter increased RNA5P expression, TRI6 may represses RNA5P expression by inhibitory binding to this predicted Tri6-binding site. For TRI10 , it may repress RNA5P expression via its regulation of TRI6 . However, repression by inhibitory binding of Tri6 does not explain the low expression level of RNA5P in the wild type under DON producing conditions. Similar to antisense- TRI5 , a low-level expression of RNA5P in the wild type may be related to fine adjustment of trichodiene synthase activities to avoid excessive DON or DON toxicity in F. graminearum . Although lncRNAs have a broad range of mode of actions [35] , [36] , transcriptional regulation of neighboring protein-coding genes is one of the common mechanisms for lncRNAs [37] . In this study, we showed that deletion of RNA5P by replacing the TRI5 promoter with that of TRI12 resulted in a significant increase in TRI5 expression and DON production although TRI12 has a lower expression level than TRI5 . Furthermore, we showed that overexpression RNA5P ectopically with the RP27 promoter had no effect but overexpression of RNA5P in situ with the TrpC promoter reduced TRI5 expression and DON production. In addition, when the Tri6-binding site in the RNA5P promoter region was mutagenized, the expression of RNA5P was significantly increased but TRI5 expression and DON production were suppressed. These results indicated that RNA5P has a cis -acting inhibitory effect on the transcription of TRI5 , which is essential for DON biosynthesis. TRI6 may regulate the expression of TRI5 by binding with the RNA5P promoter region upstream of TRI5 . The putative Tri6-binding site (GTGA/TCAC repeats separated by 0 to 8 nucleotides) is present in the promoter region of TRI5 in both F. culmorum and F. sporotrichioides although at different positions. To our knowledge, RNA5P is the first lncRNA known to regulate secondary metabolism in filamentous fungi. In yeast, plants, and animals, some cis -acting lncRNAs mediate gene silencing through the recruitment of polycomb repressive complex 2 (PRC2), while others repress the transcription of target genes by nucleosome rearrangements or formation of RNA-DNA [38] , [39] . In F. graminearum , RNA5P is transcribed from the promoter region of TRI5 . The expression of RNA5P lncRNA may inhibit the transcription of TRI5 by causing repositions of nucleosomes or the formation of RNA-DNA triplexes at its transcription initiation sites. It is also possible that RNA5P suppresses TRI5 expression by recruiting PRC2 known to be important for repressing TRI genes and other secondary metabolite gene clusters [40] to the promoter region of TRI5 . Therefore, further characterizations are necessary to determine the molecular mechanism of cis -acting regulation of TRI5 expression by RNA5P in F. graminearum . Strains and cultural conditions The wild type and mutant strains [33] and transformants generated in this study (Supplementary Table 1 ) were routinely cultured on potato dextrose agar (PDA) plates. PDA cultures incubated at 25 o C for three days were used to examine growth rate and colony morphology [41] . Conidiation and conidium morphology were assayed with conidia harvested from 5-day-old carboxymethyl cellulose (CMC) cultures [42] . To assess defects in sexual reproduction, aerial hyphae of 5-day-old carrot agar cultures were pressed down with sterile 0.1% Tween 20 and then incubated at 25 °C under black light. Perithecium formation was examined 7 days after induction for sexual reproduction [43] . PEG-mediated transformation of protoplasts was performed for gene replacement [42] . Hygromycin B (H005, MDbio, China) and geneticin (345810, Sigma-Aldrich, USA) were added to the final concentration of 300 and 150 μg/ml, respectively, for transformation selection. Plant infection and DON production assays Conidia were collected from 5-day-old CMC cultures and resuspended to a final concentration of 10 5 spores/ml in sterile distilled water. For each wheat head of cultivar Xiaoyan 22, the fifth spikelet from the bottom was drop-inoculated with 10 μl of conidium suspension. Wheat heads that underwent inoculation were covered with plastic bags for 48 hours to maintain moisture. Subsequently, the examination of infected wheat heads for diseased spikelets was conducted at 14 days post-inoculation (dpi) to determine the disease index, quantifying the number of diseased spikelets per head [44] , [45] . For assaying DON production, conidia were resuspended to a final concentration of 10 4 conidia/ml in LTB medium [46] . After incubation for 7 days, DON was measured by GCMS-QP2010 system with AOC-20i autoinjector (Shimadzu Co. Japan) [47] , [48] . For each strain, mean and standard deviation were calculated with data from three biological replicates. Generation of the TRI6 AD , TRI5 Δpromoter , tri6 , tri10 mutant alleles and transformants To generate the TRI6 AD allele deleted of the 185-bp putative promoter region of antisense- TRI6 with the split marker approach [49] , 1-kb each of its upstream and downstream fragments was amplified with the primer pairs indicated in Fig. 2c and ligated to the 5’- and 3’- terminal regions of the hygromycin phosphotransferase ( hph ) cassette fused with the thymidine kinase (TK) by overlapping PCR. The fused hph -TK selectable marker is suitable for selection for resistance against hygromycin and sensitivity to 5-fluoro-2’-deoxyuridine (Floxuridine) in fungi [50] , [51] . The resulting PCR products were transformed into protoplasts of PH-1 to isolate transformants resistant to hygromycin and screen for TRI6 AD mutants by PCR for the deletion of the 185-bp region of TRI6 . Similar approaches were used to generate transformants deleted of the promoter of TRI5 ( TRI5 Δpromoter ) as indicated in Supplementary Fig. 6 . To generate the tri6 mutant (AT6) by replacing the TRI6 gene with a reverse-transcribed hph cassette, its upstream and downstream fragments were amplified with the primer pairs indicated in Supplementary Fig. 2 and ligated to the 3’- and 5’- terminal regions of the hygromycin phosphotransferase ( hph ) cassette by overlapping PCR. The resulting PCR products were transformed into protoplasts of PH-1 to isolate transformants resistant to hygromycin and screen for the tri6 mutants by PCR. Similar approaches were used to generate the tri10 deletion mutant (AT10). All the primers used are listed in Supplementary Data 3 . Generation of the TRI6 ME , TRI5 M6B and RNA5P M mutants To generate the TRI6 ME allele, the GT-AG to AT-TG mutations were introduced by overlapping PCR with mutations in the primers. The resulting mutant allele were fused with flanking sequences of TRI6 amplified with primer pairs T6Y-1F/MER and MEF/T6Y-4R and transformed into protoplasts of TRI6 AD transformant. Transformants resistant to 25 μg/ml floxuridine (HY-B0097, MCE, USA) were isolated and screened by PCR for the replacement of hph -TK with the TRI6 ME allele by homologous recombination [50] , [51] . For TRI5 M6B , the GTGA to TGAG mutation at −1482 to −1479 was introduced by overlapping PCR with mutations in the primer pairs indicated in Fig. 8a . The resulting TRI5 M6B fragment was then fused with flanking sequences of TRI5 and transformed into protoplasts of the TRI5 Δpromoter mutant T5P. 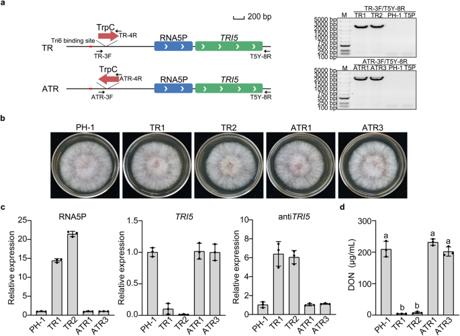Fig. 7: In situ overexpression of RNA5P with the TrpC promoter inhibitsTRI5expression. aInsertion of the TrpC promoter in the forward and reverse directions upstream from RNA5P. Red box marks the Tri6-binding site (left panel). PCR products amplified with primer pairs TR-3F/T5Y-8R and ATR-3F/T5Y-8R from genomic DNA of the wild-type strain PH-1,TRI5Δpromotertransformant (T5P), and the resulting transformants (right panel). The TrpC promoter was successfully inserted upstream of the RNA5P to generate the resulting transformants TR1 and TR2, and the insertion of TrpC-inverted promoter upstream of the RNA5P was verified by PCR in the transformants ATR1 and ATR3. Genomic DNA isolated from the wild-type PH-1 and T5P was used as a control. M, molecular marker. The experiment was repeated three times independently with similar results.bThree days PDA cultures of the wild type (PH-1), PTrpC-RNA5P mutants (TR1 and TR2), and PTrpC-invertedtransformants (ATR1 and ATR3).cRelative expression levels of RNA5P,TRI5, and antisense-TRI5were assayed by qRT-PCR with RNA samples isolated from LTB cultures of the wild type (PH-1), PTrpC-RNA5P mutants (TR1 and TR2), and PTrpC-Inverted-RNA5P transformants (ATR1 and ATR3). The relative expression level in PH-1 was arbitrarily set to 1.dDON production in LTB cultures of the same set of strains. Forcandd, mean and standard deviation were estimated with data from three (n= 3) independent replicates (marked with black dots on the bars). For DON production, different letters indicate significant differences based on one-way ANOVA followed by Turkey’s multiple-range test. Differences were considered statistically significant whenp-value is <0.05. The exactp-values are shown in the Source Data file. 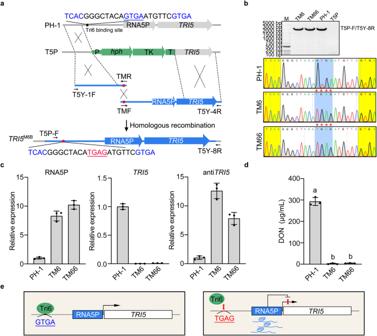Fig. 8: The GTGA to TGAG mutation in the promoter of RNA5P affects its expression and DON biosynthesis. aSchematic drawing of the genomic region of RNA5P and the gene replacement event to introduce the GTGA (underlined) to TGAG mutation at the Tri6-binding site in its promoter. The overlapping PCR products amplified with labeled PCR primers containing the TCACGGGCTACATGAGATGTTCGTGA sequence were transformed into theTRI5Δpromotertransformant (T5P) to generate theTRI5M6Btransformants carrying the GTGA to TGAG mutation. P, TrpC promoter; T, CaMV ployA signal terminator.bThe expected sizes of fragments could be amplified with primer pairs T5P-F and T5Y-8R from genomic DNA of the wild type and two independentTRI5M6Btransformants (TM6 and TM66), but not the T5P strain (upper panel). M, molecular marker. The GTGA-to-TGAG mutation in TM6 and TM66 strains was verified by Sanger sequencing of the PCR products (lower panel). The mutations are marked with red stars. The experiment was repeated three times independently with similar results.cRelative expression levels of RNA5P,TRI5, and antisense-TRI5in LTB cultures of PH-1 (arbitrarily set to 1) and two independentTRI5M6Btransformants (TM6 and TM66) carrying the GTGA to TGAG mutation.dDON production in LTB cultures of PH-1 and two independentTRI5M6Btransformants (TM6 and TM66).eA proposed model for the role of Tri6-binding on RNA5P expression. In the wild type, binding of Tri6 is inhibitory to RNA5P expression, leading toTRI5expression under DON-producing conditions. In the mutant with the GTGA-to-TGAG mutation that eliminates Tri6-binding, elevated RNA5P expression results in the suppression ofTRI5expression. Forcandd, mean and standard deviation were estimated with data from three (n= 3) independent replicates (marked with black dots on the bars). For DON production, different letters indicate significant differences based on one-way ANOVA followed by Turkey’s multiple-range test. Differences were considered statistically significant whenp-value is <0.05. The exactp-values are shown in the Source Data file. Floxuridine-resistant transformants were isolated and screened for the replacement of hph -TK with TRI5 M6B . Similar approaches were used to generate the RNA5P M transformant which has an adenine (A) insertion in the RNA5P as indicated in Fig. 4e . All the primers used were listed in Supplementary Data 3 . Generation of P TRI12 - TRI5 , P TrpC -RNA5P and P TrpC-inverted -RNA5P transformants To replace the promoter of TRI5 with that of TRI12 , a fragment containing the TRI12 promoter region was amplified with primer pairs indicated in Fig. 5b and fused to the upstream or downstream flanking sequences of TRI5 by overlapping PCR. The resulting PCR products were transformed into protoplasts of the TRI5 Δpromoter mutant T5P. Transformants resistant to floxuridine were isolated and screened by PCR for the replacement of hph -TK with TRI5 promoter. To generate the P TrpC -RNA5P transformants, the TrpC promoter was fused with the upstream and downstream flanking sequences of RNA5P amplified with primer pairs T5Y-1F/TR-2R, TR-5F/T5Y-4R by overlapping PCR. The resulting PCR products were transformed into the TRI5 Δpromoter mutant T5P. Transformants resistant to floxuridine were isolated and verified for the integration of P TrpC -RNA5P at TRI5 . Similar approaches were used to generate P TrpC-inverted -RNA5P transformant in which the TrpC promoter is in the opposite direction of RNA5P transcription. All the primers used were listed in Supplementary Data 3 . Generation of P RP27 -RNA5P and P RP27 -antisense- TRI5 constructs and transformants The yeast gap repair approach [52] was used to generate the andP RP27 -RNA5P and P RP27 -antisense- TRI5 constructs. For RNA5P, it was amplified with primer pair LT1F/LT2R and fused with the CaMV ployA signal terminator [53] amplified with primer pair LT3F/LT4R. The resulting PCR product was co-transformed with Xho I-digested pFL2 (geneticin resistance) into yeast strain XK1-25 [54] . The recombined P RP27 -RNA5P construct was rescued from Trp+ transformants and transformed into PH-1 after verification by sequencing. Transformants resistant to geneticin were isolated and verified by PCR for the integration of P RP27 -RNA5P ectopically. For antisense- TRI5 , a 299-bp fragment corresponding to 449-747 bp of the TRI5 sense transcript was amplified with primer pair SF1/SR2. The resulting PCR product was closed into pFL2 by gap repair as outlined above. The P RP27 -RNA5P construct was verified by sequence analysis and transformed into protoplasts of PH-1. Geneticin-resistant transformants were isolated and verified by PCR for the integration of P RP27 -antisense- TRI5 ectopically. All the primers used were listed in Supplementary Data 3 . Stranded RNA-seq analysis Total RNAs were isolated from hyphae harvested from 3-day-old LTB cultures with the TRIzol reagent for RNA-seq analysis (15596018, Invitrogen, USA). Conidia used to inoculate LTB were collected from 5-day-old CMC cultures. Strand-specific RNA-seq libraries constructed with the NEB Next Ultra Directional RNA Library Prep Kit (E7765, NEB, USA) were sequenced with Illumina HiSeq 2500 at Novogene Bioinformatics Technology (China). The resulting RNA-seq reads were mapped onto the updated version (Named YL1) of the reference genome of F. graminearum strain PH-1 [55] by HISAT2 [56] and visualized with the Integrative Genomics Viewer (IGV) tool (software.broadinstitute.org/software/igv/) [55] . The number of reads (count) mapped to each gene was calculated by feature Counts [57] . Genes with log 2 FC greater than 1 and FDR less than 0.05 [58] were identified as Differentially Expressed Genes (DEGs) using the edge Run package with the exact Test function. GO enrichment analysis was analyzed with Blast2GO [59] . Data from two independent biological replicates were used for differential expression analysis. The RNA-seq data generated in this study have been deposited in the NCBI Sequence Read Archive database under accession code PRJNA1044545. The reference genome of F. graminearum strain PH-1 [55] used in this study is available in the NCBI GenBank database under accession code PRJNA782099. Quantitative reverse transcription-polymerase chain reaction (qRT-PCR) assays Total RNA of each strain was isolated from 3-day-old LTB cultures with TRIzol for qRT-PCR assay (Invitrogen, USA). Conidia used to inoculate LTB were collected from 5-day-old CMC cultures. First-strand cDNA was synthesized with Fast Quant RT Kit (KP1116, TIANGEN, China) before performing qRT-PCR assays with the CFX96 Real-Time System (Bio-RAD, USA) [60] . Primer pairs for amplifying RNA5P, TRI5 , antisense- TRI5 , TRI6 , antisense- TRI6 , TRI10 , and TRI12 are 5PRT1/5RPT2, TF1/TR2, AF3/AF4, T6RTF/T6RTR (for both TRI6 and antisense- TRI6 ), T10RTF/T10RTR and T12RTF/T12RTR, respectively. The ACTIN gene (FG4G14550) was used as the internal control [28] . The relative expression level of individual genes or transcripts was calculated by the 2 –ΔΔCt method [61] . Data from three independent biological replicates were used to calculate the mean and standard deviation. All the primers used were listed in Supplementary Data 3 . Western blot analysis with the RNA5P-3×FLAG transformants To generate the P RP27 -RNA5P-3×FLAG-T CaMV construct by yeast gap repair [52] , the RNA5P-3×FLAG fusion construct was generated by PCR amplification with primers pair LT1F/L3F-R and fused with the CaMV ployA terminator [53] by overlapping PCR. The resulting PCR product was co-transformed with Xho I-digested pFL2 into yeast strain XK1-25 [54] . The recombined P RP27 -RNA5P-3×FLAG-T CaMV construct was rescued from Trp+ transformants and transformed into PH-1 after verification by sequencing. Transformants resistant to geneticin were screened by PCR. Total proteins were isolated from the resulting transformants with hyphae harvested from 3-day-old LTB cultures. For western blot analyses, total proteins were separated on 12.5% SDS-PAGE gels and transferred to nitrocellulose membranes [54] . The primary anti-FLAG antibody (F9291, Sigma, USA) and secondary anti-Mouse antibody (DY60203, DEEYEE, China) were used to detect the expression of RNA5P-3×FLAG fusion proteins. Detection with a primary anti-Tub2 β-tubulin antibody (HA720035, HUABIO, China) [62] and secondary anti-Rabbit antibody (DY60202, DEEYEE, China) were used as the loading control. Proteins isolated from the ESA1 −3×FLAG transformant [28] were used as the positive control for detection with the anti-FLAG antibody. A dilution of 1:1,000 is used for primary antibodies and 1:10,000 for secondary antibodies. Reporting summary Further information on research design is available in the Nature Portfolio Reporting Summary linked to this article.